The Wilms’ tumour suppressor Wt1 is a major regulator of tumour angiogenesis and progression Angiogenesis, activation of metastasis and avoidance of immune destruction are important for cancer progression. These biological capabilities are, apart from cancer cells, mediated by different cell types, including endothelial, haematopoietic progenitor and myeloid-derived suppressor cells. We show here that all these cell types frequently express the Wilms’ tumour suppressor Wt1, which transcriptionally controls expression of Pecam-1 (CD31) and c-kit (CD117) . Inducible conditional knockout of Wt1 in endothelial, haematopoietic and myeloid-derived suppressor cells is sufficient to cause regression of tumour vascularization and an enhanced immune response, leading to decreased metastasis, regression of established tumours and enhanced survival. Thus, Wt1 is an important regulator of cancer growth via modulation of tumour vascularization, immune response and metastasis formation. Angiogenesis is considered as one important hallmark of cancer [1] . Inhibition of tumour angiogenesis has long been suggested as a therapeutic option for cancer treatment [2] , and a large number of patients benefited from treatment with inhibitors of vascular-endothelial growth factor (VEGF) [3] . However, resistance to therapies targeting VEGF [4] and selection for metastasis [5] have been described. Recent studies showed that different cell types besides endothelial cells, orchestrate tumour angiogenesis and cancer progression. Bone marrow-derived cells (for example, monocytes—macrophages and haematopoietic progenitor cells (HPCs)) promote tumour angiogenesis [6] , [7] and stimulate tumour cell dissemination and metastasis [8] . HPCs also contribute to endothelial cells and some pericytes in the tumour [1] . A fraction of myeloid cells (myeloid-derived suppressor cells, MDSCs) promotes angiogenesis and tumour progression while at the same time provides the means to evade immune destruction by suppressing T-cell activity [1] . Therefore, identification of common markers of the mentioned cell types might allow their simultaneous targeting for efficient anticancer therapy. We found earlier that the Wilms’ tumour suppressor WT1 is highly expressed in vessels of most human tumours, but not in healthy adjacent tissues [9] . WT1 encodes a zinc-finger transcription factor with crucial functions in development and has originally been identified as a tumour suppressor [10] . Owing to its overexpression in leukaemia and a variety of solid cancers, it is nowadays considered as a potential oncogene [11] and promising target for cancer immunotherapy. Clinical trials of WT1 peptide vaccination in patients with myeloid malignancies and several solid cancers resulted in positive outcomes [12] . As WT1 is expressed only in some cancer cell types, the explication for these successful interventions might also be due to extra-tumoural WT1 targeting of vascular and stromal cells implicated in tumour progression. Due to the embryonic lethality of Wt1 -mutant mice [13] , until recently it had not been possible to determine the role of Wt1 for tumour vessel formation, its impact on tumorigenesis and the resulting consequences on cancer growth, independent from its expression in cancer cells. Here, by using multiple combinations of genetic approaches and different tumour types, we determined the phenotype of Wt1-expressing cells invading tumours, and their relevance for tumour angiogenesis, progression, metastasis and survival. WT1 expression in human tumours We investigated vascular and stromal WT1 expression in a series of 80 human cancers from seven tumour types (lung, breast, ovary, colon, pancreas, prostate carcinoma and melanoma). As described, WT1 was strongly expressed in a mostly nuclear, sometimes cytoplasmic pattern in tumour vessels [9] , but also in stromal cells ( Fig. 1 ). The intensity and frequency of WT1 expression in tumour vessels and stroma were homogenous in different samples and tumour types. Vascular and stromal WT1 were independent from WT1 expression in tumour cells [14] , [15] . WT1 was not expressed in healthy adjacent tissues, indicating that WT1 marks explicitly tumour vasculature and some stromal cells. To determine the function of vascular and stromal WT1 expression for tumourigenesis in vivo , we made use of several mouse models. 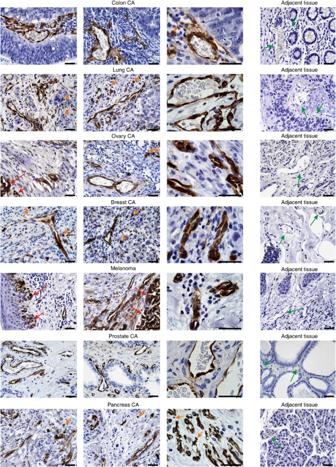Figure 1:WT1is expressed in the tumour vasculature and stromal cells of different human cancers in a homogeneous manner. Representative examples of immunostaining for WT1 (DAB substrate, brown) with haematoxylin counterstain of colon (n=14), lung (n=13), ovary (n=10), breast (n=10), prostate (n=10), pancreas (n=12) carcinoma and melanoma (n=11). For each cancer type, two examples and a higher magnification are shown. The right panel depicts healthy adjacent tissue of the respective tumour type. Red arrows point to WT1-positive tumour cells, orange arrows mark non-vascular stromal cells and green arrows mark vessels in the adjacent tissues. Note the equal degree ofWT1expression in tumour vessels and some stromal cells in different samples of the same tumour type and among the different cancer types, as well as the absence ofWT1expression in the adjacent tissues. Scale bars, 50 μm. Figure 1: WT1 is expressed in the tumour vasculature and stromal cells of different human cancers in a homogeneous manner. Representative examples of immunostaining for WT1 (DAB substrate, brown) with haematoxylin counterstain of colon ( n =14), lung ( n =13), ovary ( n =10), breast ( n =10), prostate ( n =10), pancreas ( n =12) carcinoma and melanoma ( n =11). For each cancer type, two examples and a higher magnification are shown. The right panel depicts healthy adjacent tissue of the respective tumour type. Red arrows point to WT1-positive tumour cells, orange arrows mark non-vascular stromal cells and green arrows mark vessels in the adjacent tissues. Note the equal degree of WT1 expression in tumour vessels and some stromal cells in different samples of the same tumour type and among the different cancer types, as well as the absence of WT1 expression in the adjacent tissues. Scale bars, 50 μm. Full size image Wt1 expression in the mouse To determine whether Wt1 -expressing cells similarly contribute to tumour vessels and stroma in mice, we induced syngenic B16F10 tumours (mouse melanoma cell line) in Wt1-GFP knock-in animals [16] ( Supplementary Table 1 ). Immunostaining revealed association of green fluorescent protein (GFP) with vessels and cells in the tumour stroma proving that Wt1-positive cells from the host invade the tumour. Confocal microscopy confirmed partial co-localization of GFP and Pecam-1. GFP overlapped to some extent with smooth muscle actin, desmin and CD45, indicating that Wt1 also marks other cell types than endothelial cells in the tumour stroma ( Supplementary Fig. 1 ). To investigate whether vessel-associated Wt1 is specific for tumours, we analysed GFP expression in organs of Wt1-GFP knock-in mice. GFP was detectable in kidney podocytes, the epicardium of the heart, in neurons of the brain, mesothelium of the lung, a small population of cells in the adrenal cortex, stromal cells, megacaryocytes and monocytes in the spleen and granulosa cells of the ovary. In these organs, no vascular GFP could be found. Rarely, few vessels in the heart and in brown adipose tissue were GFP positive. In contrast, in the uterus, an organ with high angiogenic capacity, a large number of vascular and stromal cells expressed GFP. We confirmed these findings by Wt1 staining of the mentioned organs ( Supplementary Fig. 2 ). Wt1 knockout reduces angiogenesis and tumour growth To determine a functional relevance of Wt1 for tumour vessel formation and tumorigenesis, we used Wt1 conditional knockout mice ( Wt1 lox/lox ) [17] crossed either with a tamoxifen-inducible Tie2-Cre [18] or VE-cadherin-Cre [19] ( Supplementary Table 1 ). Both of them have been described to be active in endothelial cells. However, Tie2 expression has also been shown in monocytic cells of haematopoietic origin, mesenchymal progenitors and MDSCs [6] , [7] , [8] , [20] . In adult Tie2-CreERT2;Wt1 lox/lox or VE-CreERT2;Wt1 lox/lox mice, Cre was activated by tamoxifen injection. Tie2-CreERT2;Wt1 lox/lox and VE-CreERT2;Wt1 lox/lox injected with vehicle and Tie2-CreERT2 mice injected with tamoxifen served as controls. We compared the effects of Wt1 loss on tumour growth in the two mouse lines by knocking out Wt1 in Tie2 + or VE-cadherin + cells, followed by subcutaneous implantation of B16 or LLC1 tumour cells. Four weeks after tumour cell injection, we determined tumour weights and vessel density in tumours. Body weights were comparable in all groups of mice (B16 tumours: Tie2-CreERT2;Wt1 lox/lox +oil 29.18±0.3 g; Tie2-CreERT2 +tamoxifen 31.91±1.17 g; Tie2-CreERT2;Wt1 lox/lox +tamoxifen 30.72±0.7 g; VE-CreERT2;Wt1 lox/lox +oil 29.5±0.45 g; VE-CreERT2;Wt1 lox/lox +tamoxifen 29.43±1.1 g; LLC1 tumours: Tie2-CreERT2;Wt1 lox/lox +oil 29.22±1.9 g; Tie2-CreERT2 +tamoxifen 28.72±1.2 g; Tie2-CreERT2;Wt1 lox/lox +tamoxifen 29.56±0.4 g; VE-CreERT2;Wt1 lox/lox +oil 26.13±0.3 g; VE-CreERT2;Wt1 lox/lox +tamoxifen 27.32±1.2 g). Tumour weights were reduced by ~90% in Tie2-CreERT2;Wt1 lox/lox +tamoxifen ( Fig. 2a,b ), and by ~50% in VE-CreERT2;Wt1 lox/lox +tamoxifen mice ( Fig. 3a,b ). Tumour growth curves revealed a comparable growth in all groups of mice at the beginning. Surprisingly, tumour volumes decreased in Tie2-CreERT2;Wt1 lox/lox +tamoxifen animals ( Fig. 2c ). After 4 weeks, we observed a combination of reduced tumour volume, lower tumour cell number, strong lymphocytic cell infiltration (arrowheads in Fig. 2e ), concentric fibrosis and central necrosis as signs of tumour regression [21] , [22] in Tie2-CreERT2;Wt1 lox/lox +tamoxifen animals. No signs of regression could be noticed in the control groups ( Fig. 2d ). When complete regression was observed, all what remained was a small scar at the injection site without presence of tumour cells. Although tumour growth became delayed in VE-CreERT2;Wt1 lox/lox +tamoxifen mice, tumours did not regress; only a slightly enhanced necrosis could be observed ( Fig. 3c,d ). 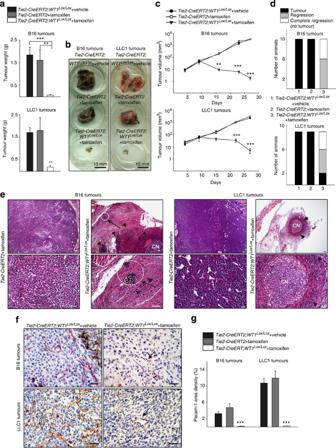Figure 2: Reduced vessel density and tumour regression uponTie2-Cre-mediated conditionalWt1knockout. (a) Quantification of tumour weights in the B16 (Tie2-CreERT2;Wt1lox/lox+tamoxifen,n=20;Tie2-CreERT2;Wt1lox/lox+vehicle,n=13;Tie2-CreERT2+tamoxifen,n=11) and LLC1 (Tie2-CreERT2;Wt1lox/lox+tamoxifen,n=11;Tie2-CreERT2;Wt1lox/lox+vehicle,n=9;Tie2-CreERT2+tamoxifen,n=8) tumour model. (b) B16 and LLC1 tumours inTie2-CreERT2;Wt1lox/lox+tamoxifen animals and control groups. Each picture shows one tumour. (c) B16 and LLC1 tumour growth curves inTie2-CreERT2;Wt1lox/lox+tamoxifen animals and respective controls. (d) Summary of the histological analysis of control animals and ofTie2-CreERT2;Wt1lox/lox+tamoxifen mice. Results were grouped as tumour, partial or complete regression. (e) haematoxylin–eosin staining of B16 and LLC1 tumours and adjacent tissues at day 27 after tumour cell injection. Note the tumour masses in control animals (left) and the small cluster of remaining tumour cells (arrows) in close proximity to large immune cell infiltrations (arrowheads) inTie2-CreERT2;Wt1lox/lox+tamoxifen animals indicating nearly complete regression. The photomicrograph of the LLC1 tumour in theTie2-CreERT2;Wt1lox/lox+tamoxifen animal represents complete regression with a remaining central necrosis (CN) surrounded by lymphocyte infiltrations (arrowheads). (f) Pecam-1 immunostaining in B16 and LLC1 tumours. (g) Quantification of Pecam-1 signal area density. Scale bars, 50 μm. Data are the mean±s.e.m. *P<0.05, **P<0.01, ***P<0.001. Figure 2: Reduced vessel density and tumour regression upon Tie2 -Cre-mediated conditional Wt1 knockout. ( a ) Quantification of tumour weights in the B16 ( Tie2-CreERT2;Wt1 lox/lox +tamoxifen, n =20; Tie2-CreERT2;Wt1 lox/lox +vehicle, n= 13; Tie2-CreERT2 +tamoxifen, n= 11) and LLC1 ( Tie2-CreERT2;Wt1 lox/lox +tamoxifen, n =11; Tie2-CreERT2;Wt1 lox/lox +vehicle, n= 9; Tie2-CreERT2 +tamoxifen, n= 8) tumour model. ( b ) B16 and LLC1 tumours in Tie2-CreERT2;Wt1 lox/lox +tamoxifen animals and control groups. Each picture shows one tumour. ( c ) B16 and LLC1 tumour growth curves in Tie2-CreERT2;Wt1 lox/lox +tamoxifen animals and respective controls. ( d ) Summary of the histological analysis of control animals and of Tie2-CreERT2;Wt1 lox/lox +tamoxifen mice. Results were grouped as tumour, partial or complete regression. ( e ) haematoxylin–eosin staining of B16 and LLC1 tumours and adjacent tissues at day 27 after tumour cell injection. Note the tumour masses in control animals (left) and the small cluster of remaining tumour cells (arrows) in close proximity to large immune cell infiltrations (arrowheads) in Tie2-CreERT2;Wt1 lox/lox +tamoxifen animals indicating nearly complete regression. The photomicrograph of the LLC1 tumour in the Tie2-CreERT2;Wt1 lox/lox +tamoxifen animal represents complete regression with a remaining central necrosis (CN) surrounded by lymphocyte infiltrations (arrowheads). ( f ) Pecam-1 immunostaining in B16 and LLC1 tumours. ( g ) Quantification of Pecam-1 signal area density. Scale bars, 50 μm. Data are the mean±s.e.m. * P <0.05, ** P <0.01, *** P <0.001. 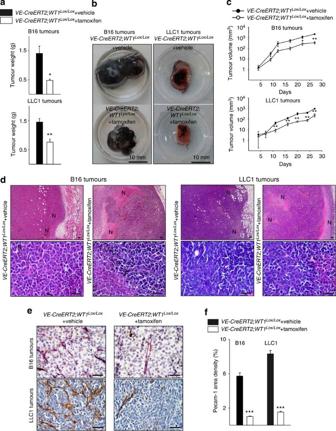Figure 3: Delayed tumour growth uponVE-cadherin-Cre-mediatedWt1knockout. (a) Quantification of tumour weights for B16 and LLC1 tumours inVE-CreERT2;Wt1lox/lox+tamoxifen mice (n=7 for each tumour type) and controls (VE-CreERT2;Wt1lox/lox+vehicle,n=7 for each tumour type). (b) B16 and LLC1 tumours inVE-CreERT2;Wt1lox/lox+tamoxifen mice and controls. (c) B16 and LLC1 tumour growth curves inVE-CreERT2;Wt1lox/lox+tamoxifen mice andVE-CreERT2;Wt1lox/lox+vehicle animals. (d) Histological aspect of B16 and LLC1 tumours. Haematoxylin–eosin staining of B16 and LLC1 tumours and adjacent tissues at day 27 after tumour cell injection. Note the larger necrotic areas (N) in tumours fromVE-CreERT2;Wt1lox/lox+tamoxifen mice compared with controls. (e) Pecam-1 immunostaining in B16 and LLC1 tumours. Note the more regular vessel architecture inVE-CreERT2;Wt1lox/lox+tamoxifen mice. (f) Quantification of Pecam-1 signal area density. Scale bars, 50 μm. Data are the mean±s.e.m. *P<0.05, **P<0.01, ***P<0.001. Full size image Figure 3: Delayed tumour growth upon VE-cadherin-Cre -mediated Wt1 knockout. ( a ) Quantification of tumour weights for B16 and LLC1 tumours in VE-CreERT2;Wt1 lox/lox +tamoxifen mice ( n =7 for each tumour type) and controls ( VE-CreERT2;Wt1 lox/lox +vehicle, n= 7 for each tumour type). ( b ) B16 and LLC1 tumours in VE-CreERT2;Wt1 lox/lox +tamoxifen mice and controls. ( c ) B16 and LLC1 tumour growth curves in VE-CreERT2;Wt1 lox/lox +tamoxifen mice and VE-CreERT2;Wt1 lox/lox +vehicle animals. ( d ) Histological aspect of B16 and LLC1 tumours. Haematoxylin–eosin staining of B16 and LLC1 tumours and adjacent tissues at day 27 after tumour cell injection. Note the larger necrotic areas (N) in tumours from VE-CreERT2;Wt1 lox/lox +tamoxifen mice compared with controls. ( e ) Pecam-1 immunostaining in B16 and LLC1 tumours. Note the more regular vessel architecture in VE-CreERT2;Wt1 lox/lox +tamoxifen mice. ( f ) Quantification of Pecam-1 signal area density. Scale bars, 50 μm. Data are the mean±s.e.m. * P <0.05, ** P <0.01, *** P <0.001. Full size image Vessel density in tumours was determined by immunostaining for Pecam-1. In both tumour models, vessel density was significantly reduced in Tie2-CreERT2;Wt1 lox/lox +tamoxifen animals ( Fig. 2f,g ). Also in VE-CreERT2;Wt1 lox/lox +tamoxifen mice, tumour vessel density was diminished, albeit to a lesser extent ( Fig. 3e,f ). To exclude that the observed differences between the two Cre lines were due to variations in Wt1 deletion, recombination efficiency was analysed, which did not evidence major differences ( Supplementary Fig. 3a ). We further investigated Wt1 levels in endothelial cells by quantitative reverse transcription (qRT)–PCR after VE-cadherin (CD144) labelling and subsequent fluorescence-activated cell sorting (FACS) from tumours of Tie2- and VE-CreERT2;Wt1 lox/lox animals. Wt1 was equally reduced in endothelial cells from both Cre lines upon knockout by tamoxifen ( Supplementary Fig. 3b ). To further confirm that the observed phenotype differences between the two Cre lines were not due to different deletion efficiencies, Tie2-CreERT2;mTmG and VE -CreERT2;mTmG reporter mice [23] were generated ( Supplementary Table 1 ). They allow lineage analysis as they express GFP following tamoxifen-induced recombination. GFP/Pecam-1 double-labelling of induced LLC1 tumours revealed that tumour vessels were to the same extent Tie2- or VE-cadherin-Cre dependent ( Supplementary Fig. 3c ). This was also reflected by a high Pecam-1/GFP overlap correlation coefficient, which showed no difference between the two Cre lines used ( Supplementary Fig. 3d ). However, in the tumours of Tie2-CreERT2;mTmG +tamoxifen animals, frequently GFP + cells could be observed, which were Pecam-1 negative, indicating that not all Tie2-Cre-dependent cells were endothelial, as further confirmed by a lower GFP/Pecam-1 overlap correlation coefficient for the Tie2-CreERT2;mTmG +tamoxifen than the VE -CreERT2;mTmG +tamoxifen-derived tumours ( Supplementary Fig. 3c,d ). Wt1 knockout increases anti-tumour immune responses Next, we confirmed an increased immune infiltration in Tie2-CreERT2;Wt1 lox/lox +tamoxifen tumours by CD3 T-cell labelling. B16 and LLC1 tumours of Tie2-CreERT2;Wt1 lox/lox +tamoxifen animals displayed a significantly higher CD3 T-cell infiltration while no difference in VE-CreERT2;Wt1 lox/lox +tamoxifen tumours compared with controls could be found ( Supplementary Fig. 4a ). To further discriminate between the different cell types involved in the increased immune response, we performed multiple labelling FACS analysis for CD45, CD3 (T cells), CD4, CD8, Cd19 (B cells), Nkp46 (natural killer (NK) cells) and CD69 and CD107 (activated lymphocytes) [24] , [25] , [26] . Tumours were collected 9 days after tumour induction to avoid secondary effects due to extensive tumour necrosis. FACS analysis revealed higher numbers of CD3 + , CD4 + and CD8 + T cells, and NK cells, but no for B cells. Furthermore, the fraction of activated CD8 + T cells and activated NK cells were higher in tumours of Tie2-CreERT2;Wt1 lox/lox +tamoxifen mice compared with controls ( Supplementary Fig. 4a,b,e ). In VE-CreERT2;Wt1 lox/lox +tamoxifen tumours, no significant differences with respect to immune cell infiltration and activation could be observed compared with controls ( Supplementary Figs 4b and 5c,d ). Wt1 has an angiogenic function Given the strong effects of Wt1 knockout under the Tie2-ERT2Cre (referred to as Wt1 KO afterwards) on tumour growth, we decided to analyse in more detail the underlying mechanisms and to identify Wt1-dependent cell types involved in tumour progression. FACS analysis of tumours from Wt1-GFP knock-in mice revealed that the majority of tumour-derived Wt1-GFP + cells also expressed Tie2 ( n =3, 83.7±4.0%) ( Supplementary Fig. 6a ), confirming the relevance of Tie2 -CreERT2 strain for our study. To determine the significance of Wt1 for vessel formation, we additionally performed ex vivo and in vivo angiogenesis assays. Aortic rings from Wt1 KO mice and the respective control groups ( n =3 each) were isolated and the time-dependent outgrowth of sprouts measured. Conditional knockout of Wt1 significantly inhibited aortic-ring sprouting ( Supplementary Fig. 6b,c ). As for the in vivo angiogenesis assay, we implanted Matrigel plugs, removed the plugs after 5 days and visualized vascularization by haematoxylin–eosin, trichrome Masson, Gordon reticulin staining and immunostaining for Pecam-1. Quantification of the number of Pecam-1-positive cells and of haemoglobin content [27] revealed significantly fewer vessels and haemoglobin in Matrigel plugs from Wt1 KO animals ( Supplementary Fig. 6d–f ). Cell types, which normally express Wt1 , that is, podocytes of the kidney and epicardial cells of the heart [17] , [28] , [29] showed no histological differences upon Tie2-Cre-mediated knockout of Wt1 ( Supplementary Fig. 6g,k ), suggesting specificity of Tie2-Cre. Heart- and kidney-specific Wt1 expression was not affected ( Supplementary Fig. 6g,h,k ) and no increase in proteinurea was detectable up to 1 year after tamoxifen induction ( Supplementary Fig. 6j ). In contrast, in the uterus, vessel formation was severely reduced and Wt1 expression lost in Wt1 KO mice ( Supplementary Fig. 6g,i ). In other organs, vessel density did not seem to be affected, as we did not detect differences for Pecam-1 area density in adrenal and thyroid glands, pancreas, heart, intestine, kidney and spleen between the different groups of mice ( Supplementary Fig. 7 ). Increased hypoxia in Wt1 KO tumours As lack of vessels would diminish oxygenation and cause hypoxia, we analysed hypoxic areas in relation to vascular structures by co-immunostaining for Pecam-1 and pimonidazole. In control animals, we observed numerous tumour vessels and small hypoxic areas, whereas in tumours of Wt1 KO mice, large hypoxic areas and few Pecam-1-positive vessels were detected ( Supplementary Fig. 8a,b ). In agreement with the observed hypoxia, immunohistochemistry for Hif-1α evidenced a large number of cells with nuclear Hif-1α accumulation in Wt1 KO mice. In control tumours, only a small number of cells in the periphery of necrotic areas showed nuclear Hif-1α staining ( Supplementary Fig. 8c,d ). Confocal microscopy of Wt1/Pecam-1-immunostained tumour samples confirmed not only the diminution of vascular structures, but also the lack of Wt1 expression in the few vessels in tumours of Wt1 KO mice ( Supplementary Fig. 8e,f ). Reduced metastases and increased survival in Wt1 KO mice Next, we analysed whether conditional knockout of Wt1 might modify metastasis occurrence. In this respect, the B16 and LLC1 models are very useful as they form spontaneous metastases [30] , [31] . We investigated serial lung and liver sections of Wt1 KO mice and the respective control groups for metastases. Of note, no metastases could be detected in the B16 model in Wt1 KO mice, and also in the LLC1 model, the number of animals bearing metastases was significantly lower in this group of mice ( Fig. 4a ). In contrast, we observed no differences in metastasis formation compared with controls in the VE-CreERT2 strain. Fifty percent of control animals and 50% of VE-CreERT2;Wt1 lox/lox +tamoxifen mice had either B16 or LLC1 metastasis. In agreement with tumour regression and reduced metastases occurrence, we observed higher survival rates in Wt1 KO mice in both tumour models ( Fig. 4b ). 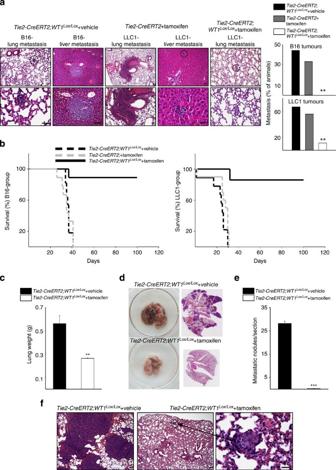Figure 4: Reduced metastasis and increased survival inWt1KO animals. (a, left panel) Representative photomicrographs of liver and lung metastasis in the three groups of mice. Metastases are indicated with a dotted green circle. Note that inTie2-CreERT2;Wt1lox/lox+tamoxifen animals no metastasis of B16 tumours occurred, and for LLC1 tumours, no liver metastasis was detectable. (a, right panel) Quantification of the percentage of animals with metastasis from B16 or LLC1 tumours, respectively. (b) Survival analyses after induction of B16 (Tie2-CreERT2;Wt1lox/lox+tamoxifen,n=17;Tie2-CreERT2;Wt1lox/lox+vehicle,n=24;Tie2-CreERT2+tamoxifen,n=22) or LLC1 tumours (Tie2-CreERT2;Wt1lox/lox+tamoxifen,n=12;Tie2-CreERT2;Wt1lox/lox+vehicle,n=11;Tie2-CreERT2+tamoxifen,n=10) indicates improved survival inWt1knockout mice compared with the control groups. (c) Quantification of lung weights 3 weeks after intravenous injection of LLC1 cells (Tie2-CreERT2;Wt1lox/lox+tamoxifen,n=5;Tie2-CreERT2;Wt1lox/lox+vehicle,n=5). (d) Lungs of control andTie2-CreERT2;Wt1lox/lox+tamoxifen animals. (e) Quantification of metastatic nodules per lung section. (f) Photomicrographs of lung metastases in controls andWt1KO animals. Note the large metastatic tumour nodules in the control compared with the micrometastasis consisting of few tumour cells in theWt1KO lung. Scale bars, 50 μm. Data are the mean±s.e.m. **P<0.01, ***P<0.001. Figure 4: Reduced metastasis and increased survival in Wt1 KO animals. ( a , left panel) Representative photomicrographs of liver and lung metastasis in the three groups of mice. Metastases are indicated with a dotted green circle. Note that in Tie2-CreERT2;Wt1 lox/lox +tamoxifen animals no metastasis of B16 tumours occurred, and for LLC1 tumours, no liver metastasis was detectable. ( a , right panel) Quantification of the percentage of animals with metastasis from B16 or LLC1 tumours, respectively. ( b ) Survival analyses after induction of B16 ( Tie2-CreERT2;Wt1 lox/lox +tamoxifen, n =17; Tie2-CreERT2;Wt1 lox/lox +vehicle, n= 24; Tie2-CreERT2 +tamoxifen, n= 22) or LLC1 tumours ( Tie2-CreERT2;Wt1 lox/lox +tamoxifen, n =12; Tie2-CreERT2;Wt1 lox/lox +vehicle, n= 11; Tie2-CreERT2 +tamoxifen, n= 10) indicates improved survival in Wt1 knockout mice compared with the control groups. ( c ) Quantification of lung weights 3 weeks after intravenous injection of LLC1 cells ( Tie2-CreERT2;Wt1 lox/lox +tamoxifen, n =5; Tie2-CreERT2;Wt1 lox/lox +vehicle, n= 5). ( d ) Lungs of control and Tie2-CreERT2;Wt1 lox/lox +tamoxifen animals. ( e ) Quantification of metastatic nodules per lung section. ( f ) Photomicrographs of lung metastases in controls and Wt1 KO animals. Note the large metastatic tumour nodules in the control compared with the micrometastasis consisting of few tumour cells in the Wt1 KO lung. Scale bars, 50 μm. Data are the mean±s.e.m. ** P <0.01, *** P <0.001. Full size image To exclude that the lower metastases formation in Wt1 KO mice was simply due to the reduced size or regression of the primary tumours, LLC1 tumour cells were intravenously injected and tamoxifen or vehicle treatment started simultaneously. After 3 weeks, lung metastases formation was studied. Lung weights in control animals were more than doubled compared with Wt1 KO mice ( Fig. 4c ). Control animals (100%) displayed large metastatic tumoural nodules invading the lung, with on average 28 tumour nodules per section. In contrast, 20% of the Wt1 KO animals had no detectable pulmonary metastasis, and the remaining 80% had on average fewer than one metastasis per section (0.23), being micrometastases, consisting of some spare tumour cells ( Fig. 4d–f ). Regression of pre-established tumours in Wt1 KO mice To investigate a potential therapeutic relevance of Wt1 inhibition for tumour treatment, we produced tumours by B16 or LLC1 cell injection in Tie2-CreERT2;Wt1 lox/lox or Tie2-CreERT2 animals prior to tamoxifen administration, which was started when the tumours reached a diameter of ~5mm and continued for 1 week ( Fig. 5 ). In Wt1 KO animals, we observed a decline of tumour volumes also when tumours were pre-established ( Fig. 5a–c ). Histological analyses showed partial or complete regression of the majority of tumours in Wt1 KO animals ( Fig. 5d,e ) and reduced metastasis occurrence ( Fig. 5f,g ). Pecam-1 immunostaining revealed a lower vessel density in Wt1 KO animals ( Fig. 5h,i ). In addition, Wt1 KO animals were resistant to a challenge of re-injection of tumour cells. To ensure that the suppression of tumourigenesis might not partially be due to ectopic tumour inoculation, we produced orthotopic lung tumours by injecting LLC1 cells into the right-lung lobe of mice. After 3 days, when a solid tumour could be detected ( Supplementary Fig. 9a ), tamoxifen or vehicle treatment was started in additional mice. After 3 weeks, lung and body weights were measured, tumour volumes determined and livers and brains analysed for potential metastases ( Supplementary Fig. 9b–h ). Tumour volumes were significantly lower in Wt1 KO mice compared with vehicle-treated controls and also lower than in untreated animals after 3 days indicating tumour regression. Histological analysis confirmed regression with increased fibrosis and lymphocyte infiltration ( Supplementary Fig. 9f vs e ). In contrast to controls, where liver metastases were detectable in 33% of the mice, no lung to liver metastases were detected in Wt1 KO animals ( Supplementary Fig. 9g,h ). 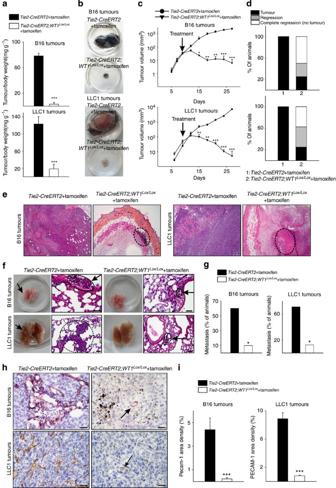Figure 5: Already established tumours regress after inducible conditional knockout ofWt1. (a) Tumour-to-body-weight ratios in controls andWt1KO animals (n=10Tie2-CreERT2;Wt1lox/loxanimals;n=10 controls for B16 tumours;n=9Tie2-CreERT2;Wt1lox/loxanimals;n=8 controls for LLC1 tumours). (b) Representative photographs of B16 and LLC1 tumours in controls andWt1KO mice. (c) B16 and LLC1 tumour growth curves inWt1KO mice and the respective controls.Wt1knockout by tamoxifen injection was started when the tumours reached a diameter of ~5 mm. (d) Summary of the histological analysis of B16 or LLC1 tumours from control animals andWt1KO mice. Results were grouped as tumour, partial or complete regression. (e) Haematoxylin–eosin staining of B16 (i) and LLC1 (j) tumours and adjacent tissue. Note the complete regression and strong lymphocyte invasion inWt1KO animals. The remaining cells in the former B16 lesion represent macrophages filled with melanin. (f) Representative photomicrographs of lung metastasis after B16 or LLC1 cell injection in conditionalWt1knockout mice and controls. Dotted circles (arrows) indicate the size of the metastatic lesion in the tissue. (g) Quantification of the number of animals with detectable metastasis from B16 or LLC1 tumours. (h) Pecam-1 immunostainings of B16 and LLC1 tumours. (i) Quantification of the area density of the Pecam-1 signal. Scale bars, 50 μm. Data are the mean±s.e.m. *P<0.05, **P<0.01, ***P<0.001. Figure 5: Already established tumours regress after inducible conditional knockout of Wt1 . ( a ) Tumour-to-body-weight ratios in controls and Wt1 KO animals ( n =10 Tie2-CreERT2;Wt1 lox/lox animals; n =10 controls for B16 tumours; n =9 Tie2-CreERT2;Wt1 lox/lox animals; n =8 controls for LLC1 tumours). ( b ) Representative photographs of B16 and LLC1 tumours in controls and Wt1 KO mice. ( c ) B16 and LLC1 tumour growth curves in Wt1 KO mice and the respective controls. Wt1 knockout by tamoxifen injection was started when the tumours reached a diameter of ~5 mm. ( d ) Summary of the histological analysis of B16 or LLC1 tumours from control animals and Wt1 KO mice. Results were grouped as tumour, partial or complete regression. ( e ) Haematoxylin–eosin staining of B16 ( i ) and LLC1 ( j ) tumours and adjacent tissue. Note the complete regression and strong lymphocyte invasion in Wt1 KO animals. The remaining cells in the former B16 lesion represent macrophages filled with melanin. ( f ) Representative photomicrographs of lung metastasis after B16 or LLC1 cell injection in conditional Wt1 knockout mice and controls. Dotted circles (arrows) indicate the size of the metastatic lesion in the tissue. ( g ) Quantification of the number of animals with detectable metastasis from B16 or LLC1 tumours. ( h ) Pecam-1 immunostainings of B16 and LLC1 tumours. ( i ) Quantification of the area density of the Pecam-1 signal. Scale bars, 50 μm. Data are the mean±s.e.m. * P <0.05, ** P <0.01, *** P <0.001. Full size image Most likely secondary to the reduced vascularization, proliferation and apoptosis were significantly affected in Wt1 KO animals. Proliferation was determined by immunostaining for proliferating cell nuclear antigen (PCNA) and apoptosis by TdT-mediated dUTP nick end labeling (TUNEL) assays. The number of PCNA-positive tumour cells was reduced in Wt1 KO animals compared with controls, whereas the number of apoptotic cells was increased ( Supplementary Fig. 10a–h ). Apoptosis was not restricted to tumour cells, but also detectable in the stroma surrounding the tumour ( Supplementary Fig. 10i–l ). Vessel regression in tumours of Wt1 KO animals To assess vessel patency and potential regression, we performed immunofluorescence double-stainings. Lectin/Pecam-1 double-labelling showed reduced Pecam-1 area density and severely compromised vessel patency in pre-established tumours followed by Wt1 knockout after 9 days, which became more pronounced after 18 days ( Fig. 6a ). At this time point, double-labelling for Pecam-1 and collagen IV to mark basement membranes confirmed blood vessel regression and persistence of some basement membrane ‘ghosts’ ( Fig. 6b ). Double-staining for Pecam-1 and desmin as markers for pericytes evidenced the remaining of some scattered pericytes in the tumours with advanced regression ( Fig. 6c ). As a potential mechanism for vessel regression, we detected a large fraction of TUNEL-positive endothelial cells in B16 and LLC1 tumours of Wt1 KO mice indicating apoptosis of endothelial cells ( Supplementary Fig. 11 ). 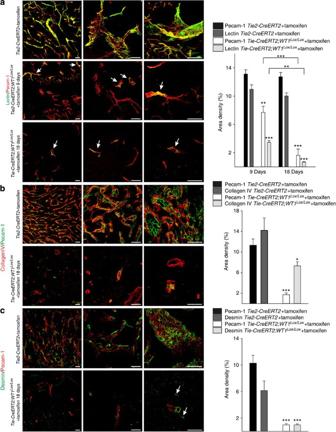Figure 6: Vessel regression inWt1KO animals. (a) Time-dependent reduction in vessel patency and vascular density uponTie2-Cre-mediated knockout ofWt1(controls,n=6;Wt1KO,n=5). Lectin staining matches Pecam-1 immunoreactivity in control animals (upper panel). Nine days after tamoxifen administration, lectin is largely reduced (arrows) indicating loss of vessel patency (middle panel). Eighteen days after tamoxifen treatment, also Pecam-1 immunoreactivity is diminished inWt1KO mice indicating vascular regression. Bar graphs show area density of Pecam-1 and lectin signals (right panel). (b) Collagen IV/Pecam-1 double-labelling shows a regular architecture of endothelial cells and basement membranes in control animals (upper panel,n=6), but remaining of only some membrane ghosts 18 days after tamoxifen treatment inWt1KO mice (lower panel,n=5). Quantification of area density of Pecam-1 and collagen IV signals is shown (right panel). (c) Pecam-1/desmin double-labelling shows close proximity between endothelial cells and pericytes in control animals (upper panel,n=6), but clear reduction of both signals and some remaining scattered pericytes (arrows) inWt1KO mice (lower panel,n=5). Quantification of area density of Pecam-1 and desmin is depicted in the bar graphs (right panel). Scale bars, 50 μm. Data are the mean±s.e.m. *P<0.05, **P<0.01, ***P<0.001. Figure 6: Vessel regression in Wt1 KO animals. ( a ) Time-dependent reduction in vessel patency and vascular density upon Tie2-Cre -mediated knockout of Wt1 (controls, n =6; Wt1 KO, n=5 ). Lectin staining matches Pecam-1 immunoreactivity in control animals (upper panel). Nine days after tamoxifen administration, lectin is largely reduced (arrows) indicating loss of vessel patency (middle panel). Eighteen days after tamoxifen treatment, also Pecam-1 immunoreactivity is diminished in Wt1 KO mice indicating vascular regression. Bar graphs show area density of Pecam-1 and lectin signals (right panel). ( b ) Collagen IV/Pecam-1 double-labelling shows a regular architecture of endothelial cells and basement membranes in control animals (upper panel, n=6 ), but remaining of only some membrane ghosts 18 days after tamoxifen treatment in Wt1 KO mice (lower panel, n =5). Quantification of area density of Pecam-1 and collagen IV signals is shown (right panel). ( c ) Pecam-1/desmin double-labelling shows close proximity between endothelial cells and pericytes in control animals (upper panel, n=6 ), but clear reduction of both signals and some remaining scattered pericytes (arrows) in Wt1 KO mice (lower panel, n=5 ). Quantification of area density of Pecam-1 and desmin is depicted in the bar graphs (right panel). Scale bars, 50 μm. Data are the mean±s.e.m. * P <0.05, ** P <0.01, *** P <0.001. Full size image Gene expression differences in Wt1 KO tumours To identify molecular events involved in the observed phenotype, we collected tumours when the size started to diminish in the Wt1 KO groups and performed qRT–PCRs on whole-tumour lysates for several genes involved in angiogenesis, apoptosis, epithelial–mesenchymal transition and immune function. The Wt1-dependent anti-angiogenic molecule thrombospondin 1 (ref. 32 ) was upregulated in both, B16 and LLC1 tumours. Other known Wt1-dependent pro-angiogenic factors such as Ets-1 and Vegf-a [9] , [33] were either unchanged or upregulated, respectively. Consistent in both tumour types, we found upregulation of caspase 9, CD3, CD69, CD83, Il2 and Il7 receptors, Ccr7 and Icos. Pecam-1, smooth muscle α-actin, desmin, c-kit, CD11b and Ly-6G (Gr-1) were downregulated in tumours of Wt1 KO animals versus controls ( Fig. 7a,b ). As the qRT-PCR results did not only confirm the observed vessel regression, but also corroborated the enhanced immune response in Wt1 KO tumours, we next addressed the question which other Wt1-expressing cell types apart from differentiated endothelial cells are implicated in the observed inhibition of angiogenesis, enhanced tumoural lymphocyte infiltration and reduced metastasis. We generated an additional mouse line, the triple-transgenic Tie2-CreERT2;Wt1 lox/GFP line ( Supplementary Table 1 ), which allows to determine through multi-labelling FACS analyses which cell types are affected by the tamoxifen-induced Wt1 knockout. 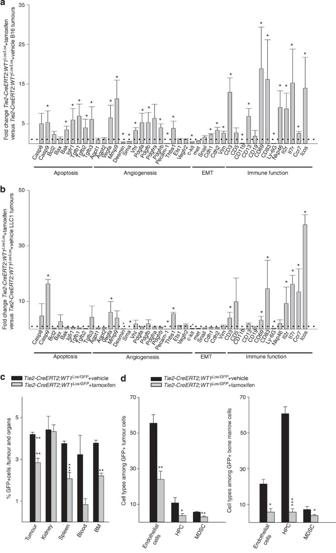Figure 7: Quantitative RT–PCR and FACS analyses corroborate additional Wt1 functions in other cell types than endothelial cells in tumours. Quantitative RT–PCR analyses of markers of apoptosis, angiogenesis, epithelial-to-mesenchymal transition (EMT) and immune function in B16 (a) or LLC1 tumours (b) ofWt1KO mice relative to controls (n=4–5 for each group). (c) FACS analysis of the fractions ofWt1-GFP-positive cells in tumours, kidney, spleen, blood and bone marrow ofWt1KO animals versus controls. (d) FACS analysis of cell types among theWt1-GFP-positive cells of the tumours (left plot, controls,n=3;Wt1KO,n=3) and the bone marrows (right plot, controls,n=3;Wt1KO,n=3). Note the reduction of GFP-positive cells in the tumours, spleens, blood and bone marrows afterWt1knockout and the significant reduction of endothelial, haematopoietic progenitor and MDSCs in the GFP-expressing cell fraction of tumours and bone marrows. Data are the mean±s.e.m. *P<0.05, **P<0.01, ***P<0.001. Figure 7: Quantitative RT–PCR and FACS analyses corroborate additional Wt1 functions in other cell types than endothelial cells in tumours. Quantitative RT–PCR analyses of markers of apoptosis, angiogenesis, epithelial-to-mesenchymal transition (EMT) and immune function in B16 ( a ) or LLC1 tumours ( b ) of Wt1 KO mice relative to controls ( n =4–5 for each group). ( c ) FACS analysis of the fractions of Wt1 -GFP-positive cells in tumours, kidney, spleen, blood and bone marrow of Wt1 KO animals versus controls. ( d ) FACS analysis of cell types among the Wt1 -GFP-positive cells of the tumours (left plot, controls, n =3; Wt1 KO, n =3) and the bone marrows (right plot, controls, n =3; Wt1 KO, n =3). Note the reduction of GFP-positive cells in the tumours, spleens, blood and bone marrows after Wt1 knockout and the significant reduction of endothelial, haematopoietic progenitor and MDSCs in the GFP-expressing cell fraction of tumours and bone marrows. Data are the mean±s.e.m. * P <0.05, ** P <0.01, *** P <0.001. Full size image Wt1 -expressing cell types in tumours In Tie2-CreERT2;Wt1 lox/GFP +tamoxifen animals, we detected a lower number of Wt1-GFP + cells in tumours, spleen, blood and bone marrow. No difference was observed in the kidneys compared with controls ( Fig. 7c ; Supplementary Fig. 12a–d ). Multi-labelling FACS was used to identify endothelial cells (CD31 + CD45 − ), HPCs (CD45 + CD31 + CD117 + Sca + ), MDSCs (CD45 + CD11b + Gr1 + ), most of which were granulocytic MDSCs (CD45 + CD11b + Gr1 + Ly6G + ), pericytes (CD45 − CD140b + ) and macrophages (CD45 + CD11b + F4/80 + Gr1 − ) among the Wt1-GFP + cells from the tumours and bone marrows. In Tie2-CreERT2;Wt1 lox/GFP +tamoxifen animals, the fractions of endothelial cells, HPCs and MDSCs were lower in tumours and bone marrows compared with controls ( Fig. 7d ; Supplementary Fig. 12e,f ). No significant changes for the fractions of pericytes (≈4%) and macrophages (≈2%) among the GFP + cells could be observed possibly reflecting the lack of Tie2-Cre activity in these cell types. Wt1 is required for MDSC function To confirm the reduction of MDSC infiltration in Wt1 KO tumours, we performed immunolabelling for Ly-6G (Gr-1), one of the principal MDSC markers. In both tumour types, Ly-6G-positive cells were significantly reduced in WT1 KO animals ( Fig. 8a ). Next, to determine the function of Wt1 expression in MDSCs, we induced LLC1 tumours in Tie2-CreERT2;Wt1 lox/lox and Tie2-CreERT2 animals, and isolated MDSCs from these tumours to knockout Wt1 in vitro by tamoxifen treatment. MDSCs isolated from the tumours of Tie2-CreERT2 animals and treated with tamoxifen served as controls to exclude unspecific tamoxifen effects. Isolated MDSCs displayed a mostly granulocytic phenotype and expressed to >90% CD11b and Ly-6G/Gr-1 ( Fig. 8b,c ). In vitro knockout of Wt1 led to a significant reduction in expression of Ly-6G/Gr1, CD11b and matrix metalloproteinase 9 (MMP9) ( Fig. 8d ). Co-culture experiments with T lymphocytes isolated from spleens of non-tumour-bearing animals revealed that KO of Wt1 in MDSCs abolished one of their major capabilities, the suppression of T-lymphocyte proliferation ( Fig. 8e,f ). This might explain the high lymphocytic infiltration observed in the Wt1 KO tumours. 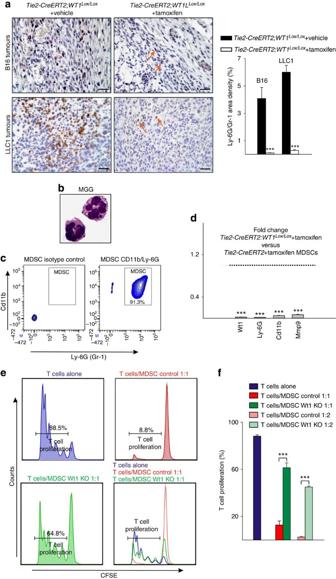Figure 8: Wt1 is important for MDSC function. (a) Ly-6G/Gr-1 immunostaining in B16 and LLC1 tumours and quantification of Ly-6G/Gr-1 signal area density. (b) Morphology of MDSCs sorted from LLC1 tumours evaluated by May-Grünwald-Giemsa staining. (c) Purity of the sorted cells for CD11b+Gr-1+ MDSCs determined by FACS. (d) Quantitative RT–PCR analyses of markers of MDSCs ofWt1KO MDSCs (derived from LLC1 tumours ofTie2-CreERT2;WT1Lox/Loxmice and tamoxifen treated for 24 hin vitro) relative to control MDSCs (derived from LLC1 tumours ofTie2-CreERT2mice and tamoxifen treated for 24 hin vitro) (n=3 for each group). (e)Wt1KO and control MDSCs were co-cultured in triplicates with CFSE-labelled CD3+ T lymphocytes isolated from spleens of non-tumour-bearing animals and proliferation assessed by flow cytometric detection of CFSE dilution after 72 h. Graphs show one representative experiment. (f) Quantification of T-cell proliferation with different T-cell/MDSC co-culture ratios. (n=3). Scale bars, 50 μm. Data are the mean±s.e.m. ***P<0.001. Figure 8: Wt1 is important for MDSC function. ( a ) Ly-6G/Gr-1 immunostaining in B16 and LLC1 tumours and quantification of Ly-6G/Gr-1 signal area density. ( b ) Morphology of MDSCs sorted from LLC1 tumours evaluated by May-Grünwald-Giemsa staining. ( c ) Purity of the sorted cells for CD11b+Gr-1+ MDSCs determined by FACS. ( d ) Quantitative RT–PCR analyses of markers of MDSCs of Wt1 KO MDSCs (derived from LLC1 tumours of Tie2-CreERT2;WT1 Lox/Lox mice and tamoxifen treated for 24 h in vitro ) relative to control MDSCs (derived from LLC1 tumours of Tie2-CreERT2 mice and tamoxifen treated for 24 h in vitro ) ( n= 3 for each group). ( e ) Wt1 KO and control MDSCs were co-cultured in triplicates with CFSE-labelled CD3+ T lymphocytes isolated from spleens of non-tumour-bearing animals and proliferation assessed by flow cytometric detection of CFSE dilution after 72 h. Graphs show one representative experiment. ( f ) Quantification of T-cell proliferation with different T-cell/MDSC co-culture ratios. ( n =3). Scale bars, 50 μm. Data are the mean±s.e.m. *** P <0.001. Full size image Wt1 transcriptionally activates Pecam-1 and c-kit To determine which of the differentially expressed genes might be directly regulated by Wt1 and be involved in the observed phenotype, we performed in silico analyses of respective promoter regions. The Pecam-1 promoter contained multiple repetitions of known Wt1-binding elements (ggagg), while the mouse c-kit promoter comprised one Wt1-binding element (gggagg) close to the transcription start site ( Fig. 9 ). To test whether Wt1 directly stimulates their activity, we cloned the promoters in a luciferase reporter vector and performed transient co-transfection experiments with Wt1(−KTS) or Wt1(+KTS) expression constructs. These two WT1 variants differ by the presence/absence of three amino acids (KTS) in the zinc-finger domain of the molecule. Pecam-1 and c-kit promoter activity was stimulated by WT1(−KTS) . In contrast, WT1(+KTS) , which has a role in post-transcriptional RNA processing and pre-messenger RNA splicing [34] , [35] rather than transcriptional regulation, did not significantly change promoter activities. Deletion of the predicted Wt1-binding sites abolished activation of these promoter constructs by Wt1(−KTS) ( Fig. 9b,f ). Chromatin immunoprecipitation assays (CHIP) using two different antibodies against Wt1 confirmed direct binding of Wt1 to the promoters, but not to 3′ untranslated region (UTR) sequences of Pecam-1 and c-kit. An antibody against acetyl-histone 3 and input DNA served as positive controls and normal rabbit serum as a negative control ( Fig. 9c,g ). Double-labelling for Wt1 and c-kit on tumours produced in C57/BL6 mice confirmed partial co-localization of Wt1 and c-kit ( Fig. 9e ). 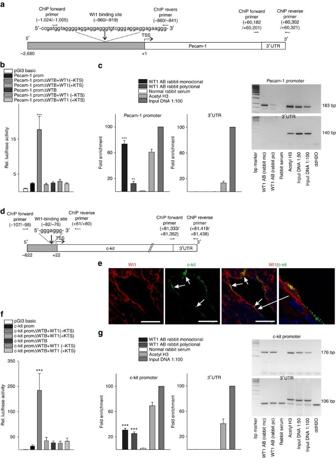Figure 9: Wt1 transcriptionally activates Pecam-1 and c-kit. Schematic representation of the putative Wt1-binding sites in the Pecam-1 (a) and c-kit (d) promoters. Positions of the cloned promoters relative to the transcription start site, positions and sequences of the putative Wt1-binding sites and positions of the oligonucleotides used for CHIP analyses are indicated. For promoter-deletion constructs, the indicated Wt1-binding sites were removed from the promoter reporter constructs. Luciferase activity of reporter constructs carrying mouse Pecam-1 promoter (b) or c-kit promoter (f) in the presence ofWt1(−KTS)orWt1(+KTS)expression constructs. Transient transfections were performed using HEK293 cells (n=12 each). The promoterless luciferase expression construct (pGl3basic) served as a negative control. ΔWTB indicates reporter constructs with deletion of the predicted Wt1-binding sites. Chromatin immunoprecipitation (ChIP,n=4) was performed in M15 cells using either monoclonal or polyclonal antibodies against Wt1 or anti-acetyl-histone H3 antibody. Normal rabbit serum served as a negative control. Input DNA was used as a positive control for quantitative PCRs (graphs on the left) or semiquantitative PCRs (representative agarose gels on the right) for the Pecam-1 promoter (c) or c-kit promoter (g) and respective 3′UTR sequences. Confocal images of double-labelled tumour sections for Wt1 and c-kit (e) revealed partial overlapping expression of both molecules within tumours. Scale bars, 50 μm. Data are the mean±s.e.m. **P<0.01, ***P<0.001. Figure 9: Wt1 transcriptionally activates Pecam-1 and c-kit. Schematic representation of the putative Wt1-binding sites in the Pecam-1 ( a ) and c-kit ( d ) promoters. Positions of the cloned promoters relative to the transcription start site, positions and sequences of the putative Wt1-binding sites and positions of the oligonucleotides used for CHIP analyses are indicated. For promoter-deletion constructs, the indicated Wt1-binding sites were removed from the promoter reporter constructs. Luciferase activity of reporter constructs carrying mouse Pecam-1 promoter ( b ) or c-kit promoter ( f ) in the presence of Wt1(−KTS) or Wt1(+KTS) expression constructs. Transient transfections were performed using HEK293 cells ( n =12 each). The promoterless luciferase expression construct (pGl3basic) served as a negative control. ΔWTB indicates reporter constructs with deletion of the predicted Wt1-binding sites. Chromatin immunoprecipitation (ChIP, n =4) was performed in M15 cells using either monoclonal or polyclonal antibodies against Wt1 or anti-acetyl-histone H3 antibody. Normal rabbit serum served as a negative control. Input DNA was used as a positive control for quantitative PCRs (graphs on the left) or semiquantitative PCRs (representative agarose gels on the right) for the Pecam-1 promoter ( c ) or c-kit promoter ( g ) and respective 3′UTR sequences. Confocal images of double-labelled tumour sections for Wt1 and c-kit ( e ) revealed partial overlapping expression of both molecules within tumours. Scale bars, 50 μm. Data are the mean±s.e.m. ** P <0.01, *** P <0.001. Full size image To determine the relevance of Wt1-dependent activation of c-kit and Pecam-1, we used as in vitro system mouse endothelial cells (C166) transduced with amphotropic virus encoding shWt1 , full-length c-kit or Pecam-1 and the corresponding control vectors. Endothelial cell c-kit expression has been described, both, in in vitro [36] and in vivo studies of human [37] and mouse [38] tissues. Western blots confirmed downregulation of Ets-1, which we already identified as a WT1 target in human endothelial cells [9] , and of c-kit and Pecam-1 upon knockdown of Wt1 ( Supplementary Figs 13a and 14 ). Wt1 knockdown decreased migration and proliferation of mouse endothelial cells, in agreement with our study on their human counterpart [9] . Overexpression of c-kit did not significantly change proliferation, but increased migration of C166 cells compared with controls. c-kit overexpression partially rescued decreased proliferation and migration upon knockdown of Wt1. Pecam-1 overexpression did neither alter proliferation nor migration compared with controls and did not rescue the Wt1 knockdown effects on these cell biological properties ( Supplementary Fig. 13b–e ). In contrast, Pecam-1 overexpression stimulated tube formation and rescued impaired tube formation of endothelial cells with Wt1 knockdown, which was also the case for overexpression of c-kit ( Supplementary Fig. 13f,g ), demonstrating that WT1 depends in part on c-kit and Pecam-1 for its pro-angiogenic functions. Lineage tracing confirms Wt1 dependency of the tumour stroma Finally, to investigate the contribution of Wt1-dependent cells to the totality of endothelial, HPCs and MDS cells present in the tumour, we performed lineage analyses using Wt1CreERT2 (ref. 39 ) crossed with mTmG mice [23] ( Supplementary Table 1 ). These animals express red fluorescence (Tomato + ) prior to, and GFP (GFP + ) following tamoxifen-inducible Wt1 -Cre-mediated recombination. Double-labelled cells signify persistence of Tomato protein after Cre-mediated recombination [23] . Therefore, double-fluorescent and single GFP + cells were combined in the analysis as Wt1 -Cre-mediated recombined and are referred to as GFP + . FACS analyses of tumour-bearing animals injected with tamoxifen revealed average fractions of 4.1%, 6.6%, 6.5% and 3.6% of GFP + cells in kidney, bone marrow, spleen and blood, respectively; the remaining cells being Tomato + . Average fractions of GFP + cells were higher in bone marrow, spleen and blood of Wt1CreERT2;mTmG +tamoxifen animals with tumours compared with healthy controls, suggesting accumulation of Wt1-dependent cell types in these organs in the presence of tumours ( Fig. 10a ). On average, 26.8% (B16 tumours) and 35.0% (LLC1 tumours) of cells represent host-derived stromal cells (Tomato + and/or GFP + ). Out of these, 58.4% and 52.0% of cells were Wt1 -Cre-mediated recombined in B16 and LLC1 tumours, respectively ( Fig. 10b,c ; Supplementary Fig. 15a–e ), pointing to the importance of Wt1 for the tumour stroma. Multi-labelling FACS analyses were performed as described on LLC1 tumours from Wt1CreERT2;mTmG +tamoxifen animals to identify individual cell types. Endothelial cells represented ~8%, HPCs ~3% and MDSCs ~5.4% of total cells in the tumour ( Fig. 10d ). On average, 59.8% of endothelial cells, 69.7% of HPCs and 72.2% of MDSCs were GFP + , indicating a major contribution of Wt1 to these cell types ( Fig. 10e ; Supplementary Fig. 15f,g ). Pericytes represented ~3% of the total number of cells, half of them being GFP + . The contribution of macrophages was highly variable between tumour samples, most of them being GFP − . 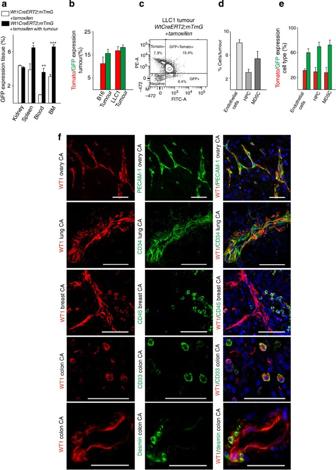Figure 10: Wt1 lineage tracing in mice and expression in human tumours. (a) FACS-based quantification of Wt1-dependent (GFP-expressing) cells in organs ofWt1CreERT2;mTmGmice after tamoxifen induction with or without tumour cell injection. Note the higher percentage of GFP+cells in bone marrow (BM), spleen and blood in tumour-bearing animals (n=3 each). (b) FACS results for B16 and LLC1 tumours (n=3 each). Wt1-dependent cells in the tumour are GFP+; non-Wt1-dependent cells from the host are Tomato positive. (c) Representative FACS example from a LLC1 tumour. (d) FACS analysis of contribution of endothelial cells, haematopoietic progenitor cells (HPCs) and myeloid-derived suppressor cells (MDSCs) to the tumour and (e) determination of the percentage of Wt1-dependent cells in each of these cell types (n=3 for B16,n=3 for LLC1). (f) Double-labelling of WT1 with Pecam-1 (endothelial cells), CD34 (endothelial, haematopoietic cells), WT1/CD45 (haematopoietic cells, MDSCs), WT1/CD33 (MDSCs) and WT1/desmin (pericytes) in human tumour samples. Scale bars, 50 μm. Data are the mean±s.e.m. *P<0.05, **P<0.01, ***P<0.001. Figure 10: Wt1 lineage tracing in mice and expression in human tumours. ( a ) FACS-based quantification of Wt1-dependent (GFP-expressing) cells in organs of Wt1CreERT2;mTmG mice after tamoxifen induction with or without tumour cell injection. Note the higher percentage of GFP + cells in bone marrow (BM), spleen and blood in tumour-bearing animals ( n =3 each). ( b ) FACS results for B16 and LLC1 tumours ( n =3 each). Wt1-dependent cells in the tumour are GFP + ; non-Wt1-dependent cells from the host are Tomato positive. ( c ) Representative FACS example from a LLC1 tumour. ( d ) FACS analysis of contribution of endothelial cells, haematopoietic progenitor cells (HPCs) and myeloid-derived suppressor cells (MDSCs) to the tumour and ( e ) determination of the percentage of Wt1-dependent cells in each of these cell types ( n =3 for B16, n =3 for LLC1). ( f ) Double-labelling of WT1 with Pecam-1 (endothelial cells), CD34 (endothelial, haematopoietic cells), WT1/CD45 (haematopoietic cells, MDSCs), WT1/CD33 (MDSCs) and WT1/desmin (pericytes) in human tumour samples. Scale bars, 50 μm. Data are the mean±s.e.m. * P <0.05, ** P <0.01, *** P <0.001. Full size image We confirmed co-expression of WT1 with markers of the above identified cell types also in human tumours. WT1 co-localized with Pecam-1 and CD34 as vascular markers, CD45 as a haematopoietic marker, CD33, which labels human MDSCs, and desmin in pericytes ( Fig. 10f ). We demonstrate here the importance of vascular and stromal Wt1 expression for tumourigenesis. In human tumour samples, we observed in a previous [9] and the present study high, homogeneous WT1 expression in the tumour vasculature and some stromal cells, independent from WT1 levels in cancer cells. This observation led us to study the functional relevance of Wt1 for tumourigenesis in vivo , using different genetically modified inducible mouse models. We confirmed the high contribution of Wt1-expressing cells to the tumour stroma in mice. To determine the relevance of Wt1 for tumour vessel formation and cancer progression, and to distinguish between the effects of a purely endothelial-specific and a broader Wt1 knockout, affecting other stromal cell types, we used Wt1 conditional knockout mice ( Wt1 lox/lox ) [17] crossed either with a tamoxifen-inducible VE-cadherin-Cre [19] or a Tie2-Cre [18] . Both Cre lines are active in endothelial cells. In addition, Tie2 expression has been shown in monocytic cells, haematopoietic progenitors and MDSCs [6] , [7] , [8] , [20] . Targeting of Wt1 in both Cre lines led to significant reduction of tumour vascularization and growth, indicating that Wt1 plays an important role for tumour progression through regulation of angiogenesis. This is in line with previous studies, where we and others demonstrated the requirement of Wt1 in coronary vessel formation during embryonic development [17] , [28] and a pro-angiogenic function of WT1 in vitro [9] . We excluded that the observed differences in the results of the Wt1 knockout with the two Cre lines were due to differing recombination efficiencies, and confirmed that Wt1 levels were equally reduced in tumour endothelial cells of both Cre lines after tamoxifen induction. We further analysed the phenotype of the Wt1 knockout under Tie2-Cre, showing that loss of Wt1 reduced angiogenesis in aortic-ring assays ex vivo and Matrigel plug assays and tumours in vivo , suggesting that both local and recruited Wt1 -expressing cells are involved in the angiogenic response. Of note, we did neither observe differences in the vascularization of most organs, nor signs of an impaired kidney function or other pathophysiological abnormalities in Wt1 KO animals. Survival analysis after tumour induction demonstrated a markedly improved survival compared with controls in the Wt1 KO animals, further excluding major pathological side effects. The sequence of reduction of tumour vessel patency, as indicated by lectin staining, followed by decreased Pecam-1 expression, appearance of basement membrane ghosts and persistence of only few Pecam-1-positive structures and scattered pericytes is in agreement with vessel regression [40] upon targeting of Wt1 . In line with the reduced vessel density, larger hypoxic areas and increased Hif-1α expression in tumours from Wt1 KO animals were observed. As Hif-1α has been shown to positively regulate Vegf [41] , it is not surprising that we detected significant increases in Vegf-a messenger RNA expression in both tumour types. We showed earlier that Wt1 is regulated by Hif-1α [42] . Wt1 in turn regulates Vegf [33] . Our data support the view that activation of the Hif-1α–Vegf axis is not sufficient to induce angiogenesis in the absence of Wt1. We did not observe changes in the expression of Wt1-regulated angiogenic Ets-1 (ref. 9 ) or its downstream target Vegfr2 (ref. 43 ) in whole-tumour lysates, which might be, as for Vegf-a, due to a high expression by the hypoxic tumour cells. In contrast, we could confirm upregulation of thrombospondin 1. Thrombospondin 1 is regarded as a key counterbalance in the angiogenic switch of tumours [1] . As Wt1 has been shown to transcriptionally suppress thrombospondin 1 (ref. 32 ), high expression of thrombospondin 1 might at least in part represent a molecular mechanism of the anti-angiogenic action upon the loss of Wt1 . The direct transcriptional activation of Pecam-1 by Wt1, which we report here, is in agreement with decreased Pecam-1 expression and reduced angiogenesis and increased endothelial cell apoptosis in tumours of Wt1 KO mice [44] . Overexpression of Pecam-1 in mouse endothelial cells knocked down for Wt1 expression partially rescued the impaired tube formation of these cells. This finding is in agreement with the literature where decreased tube formation of endothelial cells treated with antibodies against Pecam-1 has been reported [45] . Activation of c-kit by Wt1 explains the lower c-kit expression in tumours of Wt1 KO animals. c-kit is expressed by human and rodent endothelial cells [36] , [37] , [38] , and it has been shown that stem cell factor, a c-kit ligand, stimulated migration and tube formation of human endothelial cells [46] . We demonstrate here that overexpression of c-kit increases migration and tube formation of mouse endothelial cells and partially rescues the disturbed proliferation, migration and tube formation in Wt1 knockdown cells. As it is known that c-kit + HPCs contribute to tumour angiogenesis [47] , loss of Wt1 in these cells will additionally result in reduced angiogenesis. The reduced proliferation and enhanced apoptosis of tumour cells are likely due to the lower vessel density, as it is known that angiogenesis increases the rate of cancer cell proliferation [3] . Resistance of tumour cells to apoptosis has also been linked to angiogenesis and infiltrating myeloid and haematopoietic cells [48] . Interestingly, inducible Wt1 knockout under Tie2-Cre led not only to reduction of tumour growth as in the VE-Cre-mediated Wt1 knockout animals, but further to tumour regression. We could observe a higher lymphocytic tumoural infiltration in Tie2- than in VE-CreERT2;Wt1 lox/lox +tamoxifen animals. Tumours of Tie2-CreERT2;Wt1 lox/lox +tamoxifen animals displayed more CD3, CD4, CD8 and NK cell infiltration, with a higher number of activated NK and CD8 T cells compared with controls. In contrast, no differences in immune infiltration were observed in tumours of VE - CreERT2;Wt1 lox/lox +tamoxifen versus controls, suggesting that Wt1 might be expressed in Tie2-Cre-dependent cell types regulating immune cell infiltration. In addition to the strongly diminished vascularization, enhanced immune response and tumour regression in Tie2-CreERT2;Wt1 lox/lox +tamoxifen animals, we demonstrated a significantly diminished occurrence of metastasis, which was not the case for VE-CreERT2;Wt1 lox/lox +tamoxifen animals. The generation of a triple-transgenic inducible Tie2-CreERT2;Wt1 lox/GFP line allowed us to detect which cells are affected by the Wt1 knockout. In tumours, GFP + cells accounted for ~4% of total cells and the majority (~60%) were endothelial cells. Interestingly, around 10% of GFP + cells could be identified as HPCs, and 5% as MDSCs. A small number of GFP + cells were pericytes and macrophages. In the bone marrow of tumour-bearing animals, we found ~6% of GFP + cells, and, in contrast to tumours, the majority (~60%) were HPCs. Inducible knockout of Wt1 led to a significant decrease of all three cell types in tumours and bone marrow, indicating that a fraction of endothelial, HPCs and MDSCs depends on Wt1. The observed increased immune response underlines the impact of Wt1-dependent MDSCs in suppression of anti-tumour immune responses. MDSC depletion of tumours was shown to enhance therapeutic vaccination responses, leading to increased frequencies of NK, CD3, CD4 and CD8 cells invading the tumours, which became apoptotic and less metastatic [49] , a similar phenotype observed in Tie2-CreERT2;Wt1 lox/lox +tamoxifen animals. Knockout of Wt1 in MDSCs impaired their capability to suppress T-cell proliferation and might therefore explain the observed phenotype of increased immune infiltration in Wt1 KO tumours. Interestingly, MDSCs expressed less MMP9 upon Wt1 knockout. WT1 transcriptionally activates MMP9 (ref. 50 ). MMP9 secretion by MDSCs increases tumour angiogenesis and metastases occurence [51] , which could further explain the strong anti-angiogenic and anti-metastatic effect observed upon knockout of Wt1. The recent finding that WT1 transcriptionally activates TRF2 (ref. 52 ), a telomeric protein favouring angiogenesis [52] and counteracting innate immuno-surveillance of tumours [53] , provides another mechanism by which WT1 might control tumour angiogenesis and immune infiltration. Lineage analyses using Wt1CreERT2 animals [38] crossed with mTmG mice [23] corroborated the high Wt1 contribution to the tumour stroma. Around 50% of the tumour stromal cells expressed or had expressed Wt1, and further analysis showed that the majority of endothelial, HPCs and MDSCs were Wt1 dependent. We confirmed co-expression of WT1 with endothelial, HPC, MDSC and pericyte markers also in human tumour samples, suggesting a similar relevance of WT1 expression for human cancer growth. In clinical trials using WT1 peptide vaccination, apart from haematological malignancies, promising results in solid cancers were already obtained [12] . However, until now it was not recognized that inhibition of WT1 in endothelial cells, HPCs and MDSCs could contribute to these positive outcomes, which further implicates Wt1 as a critical regulator of tumourigenesis and potential therapeutic target. Antibody-mediated RNA interference [54] or antibody–drug conjugates [55] directed against WT1 might become interesting approaches for cancer therapy. Hopefully, this study may provide a cornerstone for such further developments. Animals All animals were used in accord with the French Coordination Committee on Cancer Research guidelines and local Home Office regulations (Ciepal). Wt1 lox/lox and Tie2-CreERT2 animals were crossed to generate Tie2-CreERT2;Wt1 lox/lox mice [17] , [18] . VE-cadherin-CreERT2 (ref. 19 ) mice obtained from L. Iruela-Arispe were crossed with Wt1 lox/lox animals to generate the VE-CreERT2;Wt1 lox/lox strain. Both Cre lines were backcrossed four times with C57BL6. Alternatively, Tie2-CreERT2;Wt1 lox mice were crossed with Wt1 GFP mice [16] to generate Tie2-CreERT2;Wt1 lox/GFP animals. Wt1CreERT2;mTmG animals were generated by crossing Wt1CreERT2 (ref. 38 ) (Jax stock number: 010912) with mTmG [23] (Jax stock number: 007576) mice. Age- and sex-matched Tie2-CreERT2;Wt1 lox/lox , VE-CreERT2;Wt1 lox/lox , Tie2 - CreERT2;mTmG , VE - CreERT2;mTmG and Wt1CreERT2;mTmG animals were injected for 1 week intraperitoneally (i.p.) either with sunflower oil (vehicle) or tamoxifen dissolved in sunflower oil in a dose of 33 mg kg −1 per day [56] . Tie2-CreERT2 animals injected with tamoxifen served as an additional control. Z/Pax2,CreZ/Pax2,CreZ/Pax2,Cre served as a positive control for proteinurea [56] . Male and female mice aged between 3 and 12 months were used for experiments. Deletion of Wt1 was investigated by recombination PCR as described [57] . One week after the last tamoxifen or vehicle treatment, 1 × 10 6 B16F10 or LLC1 tumour cells were injected subcutaneously. Alternatively, Matrigel plugs were produced by subcutaneous injection, or thoracic aortae were removed for aortic-ring assays. Uterus histology was investigated in synchronized mice [58] . For survival analysis, animals were kept up to 100 days after tumour production. For a ‘therapeutic approach’, tumours were produced by subcutaneous injection of B16F10 or LLC1 tumour cells and the tumours were allowed to grow until they reached a diameter of ~5 mm. Tamoxifen was injected afterwards as described above. Tumour size was measured using the caliper method [59] . Alternatively, orthotopic tumours were produced by injection of 3 × 10 4 LLC1 cells into the right-lung lobe of mice. In this case, tamoxifen injection started after 3 days. In another approach, metastases formation was investigated by intravenous inoculation of 3 × 10 5 LLC1 cells and subsequent starting of tamoxifen injections. Tumours and organs were collected after 3–4 weeks. In addition to the tumours, vessel density in adrenal glands, thyroids, pancreas, hearts, intestines, kidneys and spleens was determined by Pecam-1 immunostaining, followed by quantification of the Pecam-1 area density using ImageJ for Tie2-CreERT2 and Tie2-CreERT2;Wt1 lox/lox mice injected with tamoxifen or vehicle ( n =5 each). Wt1 GFP+/− mice were injected subcutaneously with B16F10 or LLC1 cells; tumours were collected and processed for further analyses. Age-matched female Wt1GFP +/− mice without tumours ( n =3) were used for immunohistological analysis of GFP and Wt1 expression in kidney, heart, brain, lung, intestine, liver, uterus, adrenal gland, brown adipose tissue, spleen, pancreas, muscle and ovary. Wt1CreERT2;mTmG , tamoxifen induced, Tie2-CreERT2;Wt1 lox/GFP , tamoxifen or vehicle treated, Tie2-CreERT2;Wt1 lox/lox mice, injected with tamoxifen or vehicle, and VE-CreERT2;Wt1 lox/lox mice, injected with tamoxifen or vehicle, were used for FACS analyses. LLC1 or B16 tumours, bone marrows, kidneys, spleens and blood were subjected to FACS analyses ( n =3-6). Wt1CreERT2;mTmG littermates injected with tamoxifen, but without tumours, were used as additional controls for the FACS analyses ( n= 3). Urine analysis was performed using Multistix 8SG strips (Bayer, Berkely, USA) and SDS–polyacrylamide gel electrophoresis, followed by Coomassie staining of the gels. Genotyping The genotype of animals was identified by PCR. PCR conditions and primer sequences are available on request. Cell culture B16F10 mouse melanoma cells (accession number CRL-6475) and LLC1 mouse lung cancer cells (accession number CRL-1642) were grown in Dulbecco’s modified Eagle’s medium (DMEM)-F12 medium (Lonza, Levallois-Perret, France), and C166 mouse endothelial cells (accession number CRL-2581) in DMEM medium (Lonza). M15 mouse mesonephros cells (Sigma, Lyon, France), and HEK293 cells (accession number CRL-1573) were grown in DMEM medium (Lonza). Media were supplemented with 10% fetal calf serum (FCS), 100 IU ml −1 penicillin and 100 μg ml −1 streptomycin (Invitrogen, Cergy Pontoise, France). Lentivirus production Lentivirus for transfection was prepared essentially as described [60] . pWPIR-GFP vector (8.6 μg; obtained from Didier Trono, Swiss Institute of Technology, Lausanne, Switzerland) expressing empty vector, c-kit or Pecam-1; pLKO.1 vector (8.6 μg; Sigma, St Louis, MO, USA) expressing Wt1 short hairpin RNA (Sigma) or non-coding short hairpin RNA (Sigma); or 8.6 μg of Lenti-Delta 8.91 and 2.8 μg of VSV-g were introduced into 5 × 10 6 HEK293 cells in DMEM, supplemented with 10% FCS at 37° in 5% CO 2 in 10-cm dishes, by calcium phosphate-mediated transfection. Virus containing supernatants were collected after 48 h, passed through a 0.45-μm Millipore filter and used to infect C166 cells. Detection of cell proliferation Fourty-eight hours after transduction of C166 cells, bromodeoxyuridine was added and the cells were incubated for 3 h. Afterwards, 5-bromodeoxyuridine incorporation was measured spectrophotometrically according to the manufacturer’s instructions (Millipore, Molsheim, France). Migration assays Fourty-eight hours after transduction of C166 cells, scratch migration assays [61] were performed. Images were captured after 0, 9, 20 and 27 h and scratch diameters were measured. In vitro angiogenesis assay Fourty-eight hours after transduction, C166 cells were transferred to 96-well dishes coated with 100 μl Matrigel basement membrane matrix (Chemicon, Millipore, Guyancourt, France). Branching points and tubule length were determined after additional 9 h. In vivo matrigel plug assay Matrigel (500 μl) (Becton Dickinson, Le Pont de Claix, France) containing 60 U ml −1 heparin (Sigma, Saint-Quentin Fallavier, France) were injected subcutaneously ( n =5 per group). Matrigel plugs were removed after 5 days and divided for haemoglobin quantification using Drabkin Reagent (Sigma), paraffin embedding and subsequent histological analysis. Aortic-ring assay Mice were euthanized by cervical dislocation, and thoracic aortae were removed, washed in DMEM containing antibiotics, cleaned of periadvential tissue and cut in 1-mm rings [62] . The rings were placed between two layers of 50 μl growth factor-reduced Matrigel (Becton Dickinson) supplemented with 20 U ml −1 heparin (Sigma) and overlaid with 100 μl of DMEM with VEGF (30 ng ml −1 ). Media were changed every 48 h and the number of vessels growing from each aortic ring was determined using phase-contrast microscopy. Experiments were performed in triplicates, n =3 per group. Histology and immunohistology Histology and immunohistochemistry analyses were performed according to published protocols [28] . Some animals were anaesthetized with ketamine (100 mg kg −1 i.p.) mixed with xylazine (10 mg kg −1 i.p.). Thirty minutes prior to anaesthesia, 60 mg kg −1 pimonidazole (HPI Inc., Burlington, USA) was injected i.p. to mark hypoxic areas in the tumours. Fifty μg of fluorescin isothiocyante-labelled Lycopersicon esculentum lectin (Vector Laboratories) was injected in the tail vein under anaesthesia to investigate vessel patency. After 2 min, the chest was opened and the vasculature perfused with 10 ml phosphate-buffered saline (PBS) solution containing 10 U ml −1 heparin (Sigma) via a 21-gauge cannula inserted in the left ventricle (perfusion pressure 120 mm Hg). PBS and blood exited via an incision in the right atrium. Washing with PBS was followed by fixation in 3% paraformaldehyde in PBS. Afterwards, tumours and organs were removed, embedded in OCT compound (Sakura Finetek, Villeneuve d’Ascq, France) and stored at −80 °C until cutting on a cryostat or processed for paraffin embedding. Briefly, samples from at least five different animals per group ( Tie2 -CreERT2;Wt1 lox/lox +vehicle, Tie2-CreERT2 +tamoxifen and Tie2-CreERT2;Wt1 lox/lox +tamoxifen, VE-CreERT2;Wt1 lox/lox +vehicle, VE-CreERT2;Wt1 lox/lox +tamoxifen, Wt1 GFP+/ − mice) were analysed by three independent investigators, one of them an experienced pathologist. Three-μm paraffin sections and 5-, 10-, 30- or 60-μm cryosections were used for histological and immunohistological procedures. For calculation of volumes of orthotopic lung tumours, lungs were sectioned at 3 μm and sections were stained with haematoxylin–eosin at an interval of 60 μm. The tumour area was quantified for each stained section using the ImageJ software. The tumour volume was then calculated according to: , where V i is the tumour volume, A ij the tumour area in each section and T the thickness between the sections [63] . To quantify metastasis occurrence in the subcutaneous tumour models and after intravenous injection of tumour cells, three-μm sections of the entire lung and the left lobe of the liver (only for subcutaneous tumour models) were taken at 100-μm intervals. For orthotopic tumours, metastasis was analysed in liver and brain. Haematoxylin–eosin staining was routinely performed on all tissue samples; Matrigel sections were additionally stained with Gordon reticulin and trichrome Masson. Eighty paraffin-embedded human tumour samples (lung, breast, colon, ovary, pancreas and melanoma) were used for immunohistochemical detection of WT1. The study adheres to the principles of the Declaration of Helsinki and to title 45, US Code of Federal Regulations, part 46, Protection of Human Subjects. For immunohistology, after heat-mediated antigen retrieval and quenching of endogenous peroxidase activity, antigens were detected after antibody application using the EnVision Peroxidase/DAB Detection System from Dako (Trappes, France). Sections were counterstained with haematoxylin (Sigma). For immunofluorescence double-labelling, sections were incubated with the respective antibodies after preincubation with 10% normal donkey serum in PBS with 1% bovine serum albumin and 0.1% Triton X-100. In case of primary antibodies from mouse, sections were incubated before with mouse blocking reagent (Vector Laboratories). Antigens were visualized using DyLight 488- and DyLight 594-coupled secondary antibodies derived from donkey in a 1:150 dilution (Jackson ImmunoResearch, Newmarket, Suffolk, UK). Omission of the first antibody served as a negative control. In addition, some slides were incubated with immunoglobulin G isotype controls (1:100, rabbit monoclonal, clone SP137 or 1:100, mouse monoclonal, clone MOPC-21, Abcam). The following antibodies were used: WT1 (1:100, mouse monoclonal, clone 6FH2, DAKO); PCNA (1:100, mouse monoclonal, PC10, sc-56, Santa Cruz Biotechnology, Heidelberg, Germany); PECAM-1 (CD31) (1:100, goat polyclonal, M-20, sc-1506, Santa Cruz Biotechnology), PECAM-1 (1:50, mouse monoclonal, clone JC70A, Dako), CD33 (1:100, mouse monoclonal, clone PWS44, Leica Biosystems), Pimonidazole (1:200, rabbit polyclonal, HPI Inc.), Hif1α (1:100, rabbit polyclonal, kind gift of J. Pouysségur), desmin (1:50, mouse monoclonal, clone D33, DAKO), a-smooth muscle actin (1:500, mouse monoclonal, clone 1A4, Sigma), CD34 (1:200, mouse monoclonal, clone QBEnd 10, Dako), CD45 (1:50, rat monoclonal, BD Biosciences, Le Pont de Claix, France), CD45 (1:300, mouse monoclonal, clone Ros 220, Immuntech, Marseille, France), c-kit (1:200, goat polyclonal, AF1356, R&D Systems, Lille, France), CD3 (1:100, rabbit monoclonal, clone SP7, ab16669, Abcam) and GFP (1:500, rabbit polyclonal, ab290, Abcam). Slides were viewed under an epifluorescence microscope (DMLB, Leica, Germany) connected to a digital camera (Spot RT Slider, Diagnostic Instruments, Scotland). For confocal microscopic examination (ZEISS LSM Exciter microscope, Zeiss, Jena, Germany), 3-μm paraffin sections and 30- or 60-μm cryosections were used. High-resolution Z-stacks (1, 0.7 and 0.5 μm) and three-dimensional surface rendering of Z-stacks were generated using the Zen program (Zeiss). Area densities for all immunohistological stainings were determined using the ImageJ software. Vessel area density was analysed on at least five different sections of tumours or organs per mouse, in case of paraffin sections, obtained at an interval of 200 μm, for thick cryosections, obtained with cutting intervals of 60 μm. Rarely, intervals had to be shortened due to extreme tumour regression. The extent of GFP/Pecam-1 co-localization in tumours of Tie2 -CreERT2;mTmG +tamoxifen and VE -CreERT2;mTmG +tamoxifen mice was calculated for confocal images using ImageJ, with the JACoP plugin measuring Pearson k1 and k2 coefficients on threshold-corrected images [64] . TUNEL labelling of apoptotic cells Apoptotic cells were detected by TUNEL staining of paraffin sections using the In Situ Cell Death Detection Kit (Roche Molecular Biochemicals, Meylan, France) as described previously [28] . FACS analysis Tissues (tumours, spleens, kidneys, bone marrows or blood) were minced and single-cell suspensions were obtained after enzymatic digestion (1 mg ml −1 collagenase A and 100 IU ml −1 type I DNase (Roche Diagnostics) for 1 h at 37 °C under agitation in serum-free DMEM medium. The single-cell suspension was filtered through a 70-μm cell strainer (BD Biosciences) and cells were washed twice in 2% FCS and 0.5 mM EDTA in PBS. After 15 min of saturation in Fc Block (2.4G2) from BD Biosciences, single-cell suspensions were surface stained for 40 min on ice in the dark with the following conjugated antibodies or corresponding isotype controls: anti-CD117 (2B8), anti-CD45 (30-F11), anti-CD107a (1D4B), anti-CD4 (GK1.5), anti-CD3 (145-2C11), anti-CD69 (H1.2F3) and anti-NKp46 (29A1.4) from BD Biosciences; anti-CD140b (APB5), anti-CD202b (Tek4) and anti-CD31 (390) from eBioscience (Paris, France); and anti-CD11b (M1/70), anti-F4/80 (BM8), anti-Ly-6A/E (Sca-1, D7), anti-Gr-1 (RB6-8C5), anti-Ly6G (1A8), anti-CD8 (53-6.7), anti-CD19 (6D5) and anti-CD144 (VECD1) from BioLegend (London, UK). Cells were washed with PBS containing 2% FCS and 0.5 mM EDTA. Staining was assessed with a FACSAria cytometer, and flow cytometry data were analysed using FacsDiva 6 software and FlowJo (BD Biosciences). MDSC function assays MDSCs were isolated from LLC1 tumours of Tie2- CreERT2 and Tie2 -CreERT2; Wt1 lox/lox animals by labelling cell suspensions with anti-Ly-6G-biotinylated monoclonal antibody, followed by anti-biotin-coupled magnetic beads and sorting using LS MACS columns and the MidiMACS system (Miltenyi Biotec). The isolated cells were >90% pure for CD11b+Gr1+-expressing MDSCs as determined by flow cytometry. MDSCs were cultured in complete RPMI media containing 10 ng ml −1 granulocyte-macrophage colony-stimulating factor and treated with 4-hydroxy tamoxifen (1 μM) (Sigma) for 24 h. CD3+ cells from spleens of healthy C57/Bl6 mice were sorted from cell suspensions by flow cytometry. Cells were resuspended at 10 6 per ml and incubated with carboxyfluorescein succinimidyl ester (CFSE) (5 μM) (Molecular Probes) at 37 °C for 15 min and washed three times with complete RPMI medium. T cells were placed in triplicates into 96-well plates (2 × 10 5 per well) and activated with CD3/CD28 Dynabeads (3 μl per well) and rIL2 (10 U ml −1 ) (Life Technologies). Finally, Tie2- CreERT2+tamoxifen tumour-derived MDSCs or Tie2 -CreERT2;Wt1 lox/lox +tamoxifen tumour-derived MDSCs were co-cultured with T lymphocytes in a 2:1, 1:1 and 0:1 ratio of MDSCs to T cells. Proliferation as a surrogate marker for T-cell activation was determined by CFSE dilution after 72 h after co-culture initiation using flow cytometry. Real-time RT–PCR Total RNA was isolated from uteri, kidneys and tumours using the Trizol reagent (Invitrogen). Only tumours from conditional Wt1 knockout mice, which showed no complete regression, were included. The RNA pellet was dissolved in diethyl pyrocarbonate-treated H 2 O. First-strand complementary DNA synthesis was performed with 1 μg of total RNA using oligo(dT) primers and superscript II reverse transcriptase (Invitrogen). One μl of the reaction product was taken for real-time RT–PCR amplification (ABI Prism 7000, Applied Biosystems) using a commercial SYBR Green kit (Eurogentec, Angers, France). Primer sequences are available on request. Expression of each gene was normalized to the respective Gapdh and Rplp0 expression. SDS–polyacrylamide gel electrophoresis and western blot Total cell lysates were prepared, electrophoresed and blotted, as described in detail elsewhere [9] . The following antibodies were used: WT1, rabbit monoclonal, (1:1,000, Abcam), Ets-1, rabbit polyclonal (1:500, Santa Cruz Biotechnology), PECAM-1, goat polyclonal (1:300, Santa Cruz), c-Kit, goat polyclonal (1:2,000, R&D systems), actin, goat polyclonal, (1:500, Santa Cruz), Gapdh, goat polyclonal, (1:300, Santa Cruz). Cloning and transient transfection experiments Promoter sequences of differentially expressed genes identified by real-time RT–PCR were inspected for potential Wt1-binding sites using the Promo3 software [65] . A 2.7-kb fragment from the Pecam-1 promoter was synthesized by GenScript; the c-kit promoter was a gift by C. Nishiyama [66] . All promoter constructs were subcloned in the pGl3basic luciferase expression vector (Promega). Each promoter construct was co-transfected with Wt1(−KTS) or Wt1(+KTS) expression constructs in HEK293 cells using Fugene 6 reagent (Roche Molecular Biochemicals) ( n =12 each). HEK293 cells were chosen as they express low levels of WT1, are easy to transfect and in several instances showed the ability to recapitulate in vivo regulation [9] , [27] . Putative Wt1-binding sites were deleted from the promoter constructs using the Quik Change II site-directed mutagenesis kit (Stratagene, Agilent Technologies, Massy, France) with the following oligonucleotides: c-kit, 5′-CCCCGGGCACTAGGCAAGTGCGACC-3′, Pecam-1, 5′-GAAAAGGGAATGTTAGCTGAGCTGGGGACTGGAG-3′. Deletion constructs were again co-transfected with Wt1(−KTS) or Wt1(+KTS) expression constructs ( n= 12 each). ChIP assay ChIP assay was performed on M15 cells using the manufacturer’s instructions (Millipore) as described [67] . One microgram of the following antibodies each were used: WT1, rabbit monoclonal, (ab52933, Abcam), WT1 rabbit polyclonal (sc-192, Santa Cruz Biotechnology) and acetyl-histone H3 (06-599, Upstate). Normal rabbit serum served as a negative control and dilutions of the input sample as positive control. The following primers were used: Pecam-1 promoter, 5′-TTAGCCATCCCCTGGGTCAG-3′ (forward), 5′-TCCAGAGGTGATGGGACCTG-3′ (reverse); Pecam-1 3′UTR, 5′-CCGATTCCTGGATTGCGAGA-3′ (forward), 5′-AGCGCCTCTGAGTCTCTGTA-3′ (reverse), c-kit promoter, 5′-ttattgcagcccgagagccc-3′ (forward), 5′-TGCACTTGGGCGAGAGCTGT-3′ (reverse); c-kit 3′UTR, 5′-AGTTACCGCGCTCTGTTTGA-3′ (forward), 5′-GGTACTTAAGGGGCCACACC-3′ (reverse). PCR products were electrophoresed on 4% agarose gels. Alternatively, samples were used in quantitative PCRs ( n= 3 each). Fold enrichment was calculated from cycle threshold (CT) values relative to the input signal of each experiment set to 100%. Statistical analysis Data are expressed as means±s.e.m. Analysis of variance with Bonferroni test as post hoc test or Mann–Whitney tests were performed as indicated. Significance of metastasis occurrence was calculated for Tie2-CreERT2;Wt1 lox/lox +tamoxifen animals and individual control groups using Fisher’s exact test. A P value of <0.05 was considered statistically significant. How to cite this article: Wagner, K.-D. et al. The Wilms’ tumour suppressor Wt1 is a major regulator of tumour angiogenesis and progression. Nat. Commun. 5:5852 doi: 10.1038/ncomms6852 (2014).